The molecular network governing nodule organogenesis and infection in the model legumeLotus japonicus Bacterial infection of interior tissues of legume root nodules is controlled at the epidermal cell layer and is closely coordinated with progressing organ development. Using spontaneous nodulating Lotus japonicus plant mutants to uncouple nodule organogenesis from infection, we have determined the role of 16 genes in these two developmental processes. We show that host-encoded mechanisms control three alternative entry processes operating in the epidermis, the root cortex and at the single cell level. Single cell infection did not involve the formation of trans-cellular infection threads and was independent of host Nod-factor receptors and bacterial Nod-factor signals. In contrast, Nod-factor perception was required for epidermal root hair infection threads, whereas primary signal transduction genes preceding the secondary Ca 2+ oscillations have an indirect role. We provide support for the origin of rhizobial infection through direct intercellular epidermal invasion and subsequent evolution of crack entry and root hair invasions observed in most extant legumes. Symbiosis between legumes and rhizobia is a non-pathogenic bacterial infection of a multicellular organism. Development of nitrogen-fixing root nodules is governed by a host genetic programme that synchronizes two processes running in parallel. Nodule primordia are formed from root cortical cells that re-initiate cell division, and simultaneously a bacterial infection process targets the developing primordia. This coordination has made separation of the molecular mechanisms underlying these two very different plant developmental processes difficult and has particularly limited the assignment of the specific role of plant genes governing bacterial infection. Adding further challenges to this analysis, microscopic investigation of a variety of wild and cultivated legume species has distinguished at least three different entry modes called infection thread invasion, crack entry and epidermal infection [1] . At the cellular level, infection of model legumes Lotus japonicus (Lotus) and Medicago truncatula , as well as crops such as soybean, pea and clover, is initiated when bacteria are entrapped by a curled root hair [2] . Local cell wall hydrolysis and invagination of the plasma membrane then lead to formation of infection threads that traverse to the base of the root hair cell. These plant-derived tubular structures proceed into the root cortex, branch and ramify in the nodule primordium [2] . Finally, rhizobia colonizing infection threads are released into plant cells, in which, surrounded by a peribacteriod membrane, they reduce atmospheric dinitrogen to ammonium. Continued containment of invading bacteria within specialized plant membranes is the characteristic feature of this intracellular invasion process. Loss-of-function mutants in Lotus and M. truncatula have shown that perception of the rhizobial lipochitin-oligosaccharide (Nod-factor) [3] , [4] through Nod-factor receptors (NFR1 NFR5) [5] , [6] , [7] is required to trigger the earliest physiological responses to Nod-factor signals, Ca 2+ influx, membrane depolarization and Ca 2+ oscillations (spiking) [5] , [8] , as well as for the initiation of nodule development [5] , [6] , [7] . Domain swaps and amino-acid substitutions have further suggested that the LysM domains of NFR1 and NFR5 receptors mediate the perception of bacterial Nod-factor and that recognition depends on Nod-factor structure [9] . The downstream signalling pathway is shared with mycorrhizal symbiosis and encompasses a leucine-rich repeat receptor kinase ( SymRK) [10] , [11] , cation channels ( Castor and Pollux) [12] , [13] , [14] , nucleoporins ( Nup85 and Nup133) [15] , [16] , a calcium calmodulin-dependent protein kinase ( CCaMK ) [17] , [18] , [19] and a nuclear localized coil–coil protein ( Cyclops ) [20] . SymRK, Castor , Pollux, Nup85 and Nup133 function upstream of Ca 2+ spiking, whereas CCaMK and Cyclops were suggested to decode the Ca 2+ oscillation signature [17] , [18] , [19] . The current understanding is that the Nod-factor perceived at the plasma membrane through NFR receptors, accompanied by activation of the SYMRK receptor, leads to transmission of a secondary signal releasing calcium spiking in the nucleoplasm [21] . In turn, this calcium oscillation signature is decoded by nuclear-localized CCaMK [17] , [18] , [19] . Similarly, the nuclear membrane localization of CASTOR and POLLUX potassium channel proteins suggests a role in the regulation of calcium channels and in the release of calcium from the nuclear envelope [14] . Several alternative functions were suggested for nucleoporins, including import of secondary signal(s), anchoring of potassium channel proteins, transport of the NSP2 proteins mentioned below and regulation of calcium fluxes [15] , [16] . Further downstream of the shared pathway, putative transcriptional regulators of the NIN [22] , [23] GRAS ( Nsp1, Nsp2 ) [24] , [25] , [26] , [27] and ERF [28] , [29] families are required for upregulation of nodule-expressed genes and initiation of nodulation [30] , [31] . Formation of nodule primordia involves dedifferentiation and reactivation of cortical root cells, and both gain-of-function and loss-of-function mutants have shown that cytokinin signalling through the cytokinin receptor ( Lhk1 ) [32] , [33] is important for reactivation of the cell cycle in cortical cells. The genetic requirement for infection thread development is less well described but both the Nap1 and Pir1 genes that encode proteins of the SCAR/WAVE complex activating actin rearrangement in root hairs [34] and Cerberus , which encodes a putative E3 ubiquitin ligase [35] are required for normal infection thread progression. Mutational perturbation of most of the genes mentioned above leads to simultaneous absence of, or severe impairment of, organ formation and infection thread development. This has made the dissection of direct and indirect roles of the affected proteins within the two processes virtually impossible. Circumventing this obstacle, in this study, we have taken advantage of the two Lotus gain-of-function alleles, snf1 and snf2 , encoding a T265I calcium calmodulin-dependent kinase CCaMK [17] , [36] , [37] and a L266F cytokinin receptor LHK1 [32] , [33] , [36] respectively. These gain-of-function alleles uncouple organogenesis from infection and cause a development of empty spontaneous nodules in the absence of the bacterial symbiont, Mesorhizobium loti ( M. loti ), or bacterial Nod-factor signals. Using double, triple and quadruple mutants in the gain-of-function snf1 and snf2 genetic background, or transgenic roots, we have assigned genes and corresponding functions to separate paths or connecting cross-signalling functions in the complex molecular network controlling legume symbiosis. Altogether, the mechanistic role of 16 receptors and signal-transduction components previously characterized in a decade of gene discoveries was brought together in a synthesis defining a functional framework coordinating infection and organogenesis. Genes required for organogenesis and indirectly for infection We assumed that NFR1 and NFR5 receptors would be necessary for rhizobial infection of spontaneous nodule primordia and therefore we first investigated the effect of symrk , castor , pollux , nup133 and nup85 loss-of-function mutations on the formation and infection of spontaneous nodules. 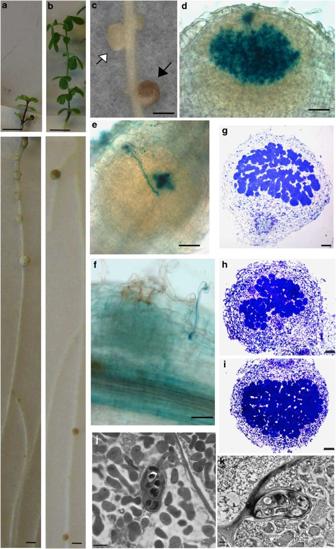Figure 1: Infection of spontaneous nodules and development of nitrogen-fixing root nodules onsymrk-3 snf1mutants. (a) Spontaneous nodules on uninoculated plant. (b) Nitrogen-fixing pink nodules onM. loti-inoculated plant. Roots are shown close-up to visualize nodules. (c) Close-up of root nodules. Closed arrow: infected pink nodule, open arrow: white uninfected nodules. (d,e) Infection of primordia visualized by staining ofM. loti::lacZbacteria within infection threads. (f) Root hair infection thread. (g) Thin section of wild-type control infected byM. loti. (h,i) Thin sections of a partly and fully infected pink nodule. (j,k) EM of infection threads inM. loti-infected nodules. Size bars: (a,b): upper (shoot) part: 1 cm; lower (root) part: 1 mm, (c): 1 mm,d–f: 20 μm,i: 200 μm,h: 100 μm,j: 1 μm,k: 1 μm. Analysis of SymRK gene function is presented in detail to illustrate the approach ( Table 1 ; Supplementary Fig. S1 online). To distinguish the role of the SYMRK receptor in infection and organogenic processes more precisely, we determined the impact of two loss-of-function non-nodulating alleles ( symrk-1 and symrk-3 ) caused by insertion of LORE retroelements [10] in an snf1 genetic background, that is, in the presence of an autoactive CCaMK [17] . First, the effect on organogenesis was scored as the ability to form spontaneous nodules and, when no change in this capacity was observed, the effect on infection was subsequently scored as the frequency of pink functional nodules among the spontaneously formed non-functional white nodules. A set of snf1 and symrk single mutants and symrk snf1 double mutants were inoculated with M. loti on nitrogen-free agar slopes. As previously reported, snf1 mutants developed fully infected nitrogen-fixing pink nodules with a high frequency, resulting in green plants and plant growth, whereas symrk mutants did not develop any nodules or nodule primordia and plants were nitrogen starved, yellow and did not grow ( Table 1a ; Supplementary Fig. S1 ). Spontaneous nodule primordia developed in symrk snf1 double mutants. Unexpectedly, these spontaneous nodule primordia were also infected by M. loti , and nitrogen-fixing nodules, rescuing the non-nodulating and nitrogen-starved phenotype conferred by symrk mutations [10] , were established ( Fig. 1a–c , Table 1a , Supplementary Fig. S1 ). The frequency of pink nodules in symrk-3 snf1 and symrk-1 snf1 double mutants was relatively high, ~20% compared with 69% in snf1 and 84% in wild type ( Table 1a ). This observation led us to determine whether the infections in symrk snf1 mutants took place through root hair infection threads, that is, whether SYMRK was dispensable for infection thread formation in the presence of autoactive snf1 CCaMK. Visualization of an M. loti strain constitutively expressing the β-galactosidase ( lacZ) reporter gene showed invasion through root hair infection threads in symrk snf1 mutants ( Figs. 1d–k and 2a–f ). However, emergence was delayed and the number was reduced (five infection threads per wild-type root versus 0, and 55 versus 8, 1 and 2 weeks after inoculation, respectively). A closer inspection revealed infection threads in root hairs in close proximity to nodule primordia, and misguided infection thread growth associated with balloon-like swellings was not unusual ( Figs. 1f and 2e–f ). Light microscopy of thin sections of pink symrk snf1 nodules shows infected cells completely or partly occupying the inner root nodule tissue ( Fig. 1g–i ) and an average of 32 trans -cellular infection threads per section compared with 28 in wild type ( Table 1a ). Confirming the light microscopy results, electron microscopy micrographs visualized infection threads in nodules with infected cells ( Fig. 1j,k ). Containment of bacteria within infection threads without release as reported in SymRK/DMI2 RNA-mediated interference lines of Sesbania and Medicago [38] , [39] was not observed, implying that signal transduction through the SYMRK receptor was dispensable for root hair infection thread formation and bacterial release in Lotus snf1 nodules. Table 1 Frequency of infected pink nodules, presence of infection threads in root hairs and trans -cellular infection threads in nodule sections. Full size table Figure 1: Infection of spontaneous nodules and development of nitrogen-fixing root nodules on symrk-3 snf1 mutants. ( a ) Spontaneous nodules on uninoculated plant. ( b ) Nitrogen-fixing pink nodules on M. loti- inoculated plant. Roots are shown close-up to visualize nodules. ( c ) Close-up of root nodules. Closed arrow: infected pink nodule, open arrow: white uninfected nodules. ( d , e ) Infection of primordia visualized by staining of M. loti::lacZ bacteria within infection threads. ( f ) Root hair infection thread. ( g ) Thin section of wild-type control infected by M. loti . ( h , i ) Thin sections of a partly and fully infected pink nodule. ( j , k ) EM of infection threads in M. loti- infected nodules. Size bars: ( a , b ): upper (shoot) part: 1 cm; lower (root) part: 1 mm, ( c ): 1 mm, d – f : 20 μm, i : 200 μm, h : 100 μm, j : 1 μm, k : 1 μm. 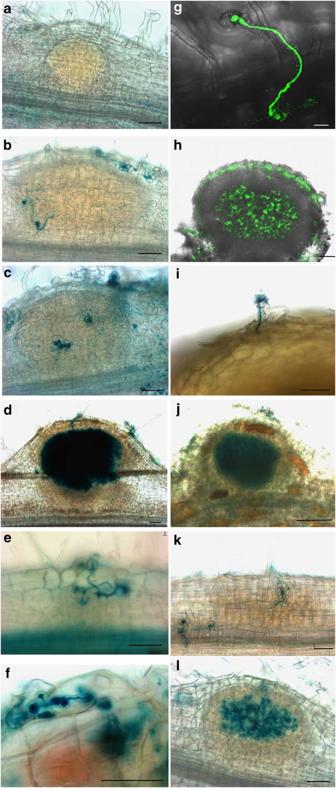Figure 2: Infection of spontaneously induced nodule primordia in double mutants. (a–f)symrk-3 snf1nodules. (a) Uninfected primordium. (b,c) Examples of bacteria in infection threads approaching a spontaneous nodule primordium. (d) Old, fully infected nodule. (e,f) Close-up of partly misguided infection threads with swellings. (g) Infection thread innup85-1 snf1root hair. (h) Fully infectednup85-1 snf1nodule. (i) Infection thread innup133-3 snf1root hair above spontaneous nodule primordium. (j) Fully infectednup133-3 snf1nodule. (k) Infection thread inL. japonicuswild-type root hair above nodule primordium. (l) Young, fully infected wild-type nodule. Infection threads and infected tissue were visualized by staining ofM.lotibacteria expressinglacZ(a–fandi–l) or by fluorescence ofM. lotibacteria expressing eGFP (g–h). Scale bars (a–g,i,k,l): 20 μm, (j): 50 μm, (h): 100 μm. Full size image Figure 2: Infection of spontaneously induced nodule primordia in double mutants. ( a–f ) symrk-3 snf1 nodules. ( a ) Uninfected primordium. ( b , c ) Examples of bacteria in infection threads approaching a spontaneous nodule primordium. ( d ) Old, fully infected nodule. ( e , f ) Close-up of partly misguided infection threads with swellings. ( g ) Infection thread in nup85-1 snf1 root hair. ( h ) Fully infected nup85-1 snf1 nodule. ( i ) Infection thread in nup133-3 snf1 root hair above spontaneous nodule primordium. ( j ) Fully infected nup133-3 snf1 nodule. ( k ) Infection thread in L. japonicus wild-type root hair above nodule primordium. ( l ) Young, fully infected wild-type nodule. Infection threads and infected tissue were visualized by staining of M.loti bacteria expressing lacZ ( a – f and i – l ) or by fluorescence of M. loti bacteria expressing eGFP ( g – h ). Scale bars ( a–g , i , k , l ): 20 μm, ( j ): 50 μm, ( h ): 100 μm. Full size image Similar to symrk mutants, nucleoporin nup133 and nup85 mutants and potassium channel pollux and castor mutants show limited root hair responses to M. loti and lack the calcium-spiking characteristic for Nod-factor-induced signalling [8] , [12] , [13] , [14] , [15] , [16] . As previously reported, the inoculation of nup133 and nup85 mutants with M. loti resulted in a temperature-dependent non-functional and reduced infection phenotype [15] , [16] . In contrast, nup133 snf1 and nup85 snf1 double mutants were invaded through root hair infection threads and nitrogen-fixing nodules developed to rescue the ineffective nodulating phenotype of the single mutants at both the normal 21 °C growth conditions and the non-permissive 26 °C ( Table 1a ; Figs. 2g–l , 3 and 4 ; Supplementary Fig. S1 ). Infection threads were observed in root hairs in proximity to nodule primordia ( Fig. 2g–j ). Comparable infections of the non-nodulating castor and pollux mutants were observed using a dominant T265D version of CCaMK and transgenic roots generated by Agrobacterium rhizogenes- mediated transformation ( Table 1a ). 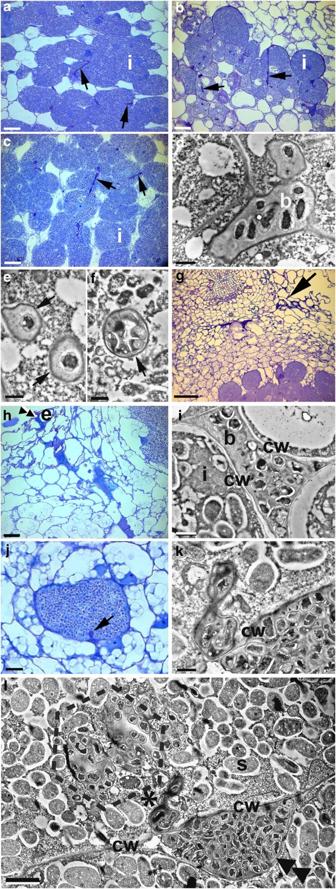Figure 3: Intercellular infection mechanisms. (a) Control showingtrans-cellular infection threads (ITs) in thin section ofM. loti-infected wild-type nodule. Arrows: ITs; (b)trans-cellular ITs (arrows) innfr1-1nfr5-2 symrk-3 snf1nodule infected byM. loti; (c)trans-cellular ITs (arrows) insymrk-3snf1infected byM. loti.(d) and (e) Transmission electron microscopy (TEM) micrograph of ITs (arrows) inM. loti-infected wild-type nodule. (f) Infection thread (arrow) inM. loti-infectednfr1-1 nfr5-2 symrk-3 snf1nodule. (g) Crack entry (arrow) ofM. lotiintonfr1-1 nfr5-2 symrk-3 snf1nodule. (h) Intercellular epidermal infection ofnodCmutant bacteria into annfr1-1 nfr5-2 snf1nodule. Double arrow: bacterial entry point. e: Epidermal cell. (i) IntercellularnodCbacteria insidenfr1-1 nfr5-2 snf1nodule. cw: Cell wall, b: bacteria. (j) Single cell infection in annfr1-1 nfr5-2 snf1nodule. Infection thread (arrow) initiated by intercellularnodCbacteria (double arrowhead). (k) Close-up of infection thread marked by a * in (l): a short infection thread initiated from an adjacent pocket of intercellularnodCbacteria in annfr1-1 nfr5-2 snf1nodule. cw: Cell wall. (l) Enlarged infection thread release structure in annfr1-1 nfr5-2 snf1nodule infected bynodC.Hexagon (dashed line) surrounds the butterfly-shaped release structure. *Infection thread, cw: cell wall, double arrowhead: pocket of intercellular bacteria, i: infected cell, s: symbiosome. Size barsa–c: 20 μm,d,i,k,l: 1 μm,e,f: 500 nm,g: 50 μm,h: 10 μm,j: 5 μm. Figure 3: Intercellular infection mechanisms. ( a ) Control showing trans -cellular infection threads (ITs) in thin section of M. loti- infected wild-type nodule. Arrows: ITs; ( b ) trans -cellular ITs (arrows) in nfr1-1nfr5-2 symrk-3 snf1 nodule infected by M. loti ; ( c ) trans- cellular ITs (arrows) in symrk-3snf1 infected by M. loti. ( d ) and ( e ) Transmission electron microscopy (TEM) micrograph of ITs (arrows) in M. loti- infected wild-type nodule. ( f ) Infection thread (arrow) in M. loti- infected nfr1-1 nfr5-2 symrk-3 snf1 nodule. ( g ) Crack entry (arrow) of M. loti into nfr1-1 nfr5-2 symrk-3 snf1 nodule. ( h ) Intercellular epidermal infection of nodC mutant bacteria into an nfr1-1 nfr5-2 snf1 nodule. Double arrow: bacterial entry point. e: Epidermal cell. ( i ) Intercellular nodC bacteria inside nfr1-1 nfr5-2 snf1 nodule. cw: Cell wall, b: bacteria. ( j ) Single cell infection in an nfr1-1 nfr5-2 snf1 nodule. Infection thread (arrow) initiated by intercellular nodC bacteria (double arrowhead). ( k ) Close-up of infection thread marked by a * in ( l ): a short infection thread initiated from an adjacent pocket of intercellular nodC bacteria in an nfr1-1 nfr5-2 snf1 nodule. cw: Cell wall. ( l ) Enlarged infection thread release structure in an nfr1-1 nfr5-2 snf1 nodule infected by nodC. Hexagon (dashed line) surrounds the butterfly-shaped release structure. *Infection thread, cw: cell wall, double arrowhead: pocket of intercellular bacteria, i: infected cell, s: symbiosome. Size bars a–c : 20 μm, d , i , k , l : 1 μm, e , f : 500 nm, g : 50 μm, h : 10 μm, j : 5 μm. 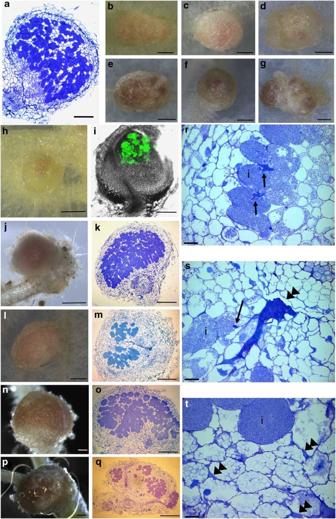Figure 4: Examples of nodule morphologies and thin sections of infected spontaneous nodules. (a) Thin section of a fully infectedM. lotinodule on ansnf1plant, (b)nfr1-1 snf1infected withM. loti, (c)nfr5-2 snf1infected withM. loti, (d)har1-3 snf1infected withnodC, (e)har1-3 snf1infected withnodA, (f)har1-3 snf1infected withnodC, (g)har1-3 snf1infected withnodC, (h)snf1infected withM. lotiexpressing eGFP, (i) fluorescence microscopy of a thin section of nodule in (h), (j)nup85-1 snf1infected withM. loti, (k) thin section of nodule in (j), (l)nfr1-1nfr5-2 snf1infected withM. loti, (m) thin section of nodule in (l), (n)nfr1-1 nfr5-2 symrk-3 snf1infected withM. loti, (o) thin section of nodule in (n), (p)nfr1-1 nfr5-2 symrk-3 snf1infected withM. loti, (q) thin section of nodule in (p), (r, s, t) thin sections of nodules ofnfr1-1 nfr5-2 symrk-3 snf1infected withM. loti. i: infected cell, double arrowheads: pockets of intercellular bacteria, arrows: infection threads, emerging from pockets. Size bars (a), (i), (k), (m), (o), (q): 200 μm; (b–h), (j), (l): 500 μm; (n) and (p): 200 μm; (r–t): 5 μm. Full size image Figure 4: Examples of nodule morphologies and thin sections of infected spontaneous nodules. ( a ) Thin section of a fully infected M. loti nodule on an snf1 plant, ( b ) nfr1-1 snf1 infected with M. loti , ( c ) nfr5-2 snf1 infected with M. loti , ( d ) har1-3 snf1 infected with nodC , ( e ) har1-3 snf1 infected with nodA , ( f ) har1-3 snf1 infected with nodC , ( g ) h a r1-3 snf1 infected with nodC , ( h ) snf1 infected with M. loti expressing eGFP, ( i ) fluorescence microscopy of a thin section of nodule in ( h ), ( j ) nup85-1 snf1 infected with M. loti , ( k ) thin section of nodule in ( j ), ( l ) nfr1-1nfr5-2 snf1 infected with M. loti , ( m ) thin section of nodule in ( l ), ( n ) nfr1-1 nfr5-2 symrk-3 snf1 infected with M. loti , ( o ) thin section of nodule in ( n ), ( p ) nfr1-1 nfr5-2 symrk-3 snf1 infected with M. loti , ( q ) thin section of nodule in ( p ), ( r, s, t ) thin sections of nodules of nfr1-1 nfr5-2 symrk-3 snf1 infected with M. loti . i: infected cell, double arrowheads: pockets of intercellular bacteria, arrows: infection threads, emerging from pockets. Size bars ( a ), ( i ), ( k ), ( m ), ( o ), ( q ): 200 μm; ( b–h ), ( j ), ( l ): 500 μm; ( n ) and ( p ): 200 μm; ( r–t ): 5 μm. Full size image Genes required for infection but dispensable for organogenesis nap1 , pir1 and cerberus mutant plants have all previously been shown to develop nodule primordia with aberrant infection thread formation or progression [34] , [35] . To extend the infection thread observations, we transformed these mutants with the T265D construct of CCaMK. The phenotype of arrested infection threads and lack of infected nodules in the mutant plants transformed with T265D CCaMK confirmed that Nap1 , Pir1 [34] and Cerberus [35] genes function in the infection thread pathway ( Table 1b ). Gene functions required for both infection and organogenesis Previous characterization of nin , nsp1 and nsp2 mutants suggests a function for these transcriptional regulators in both infection and organogenesis [22] , [23] , [24] , [25] , [26] , [27] . The lack of spontaneous nodules observed in nin-2 snf1 double mutants, as well as the unchanged phenotype of nsp1 and nsp2 mutants, transformed with the T265D CCaMK construct confirmed their role in organogenesis. Microscopy of roots inoculated with the M. loti lacZ strain detected root hair deformations but no infection threads in nin-2 snf1 double mutants ( Table 1c ). The impaired infection and organogenesis phenotype were also unchanged in the nsp1 and nsp2 mutants transformed with the T265D variant of CCaMK ( Table 1c ). Cross-talk between organogenesis and infection pathways The availability of corresponding gain-of-function ( snf1 , snf2 ) [17] , [32] and loss-of-function ( ccamk , hit1 ) [17] , [33] mutants of CCaMK and the Lhk1 cytokinin receptor genes enabled us to investigate the interdependence of organogenesis and root hair infection. Infection of reciprocal snf1 hit1 and ccamk-13 snf2 double mutants was analysed, together with symrk-3 snf1 and symrk-3 snf2 mutants. Inactivation of CCaMK in ccamk-13 snf2 resulted in an absence of infection of the spontaneously formed primordia caused by snf2 gain-of-function cytokinin receptor activity. In addition, inactivation of the SYMRK receptor in symrk-3 snf2 mutants resulted in a very low infection frequency of snf2- induced spontaneous nodules compared with the autoactive CCaMK-induced primordia in symrk-3 snf1 double mutants ( Table 1d and a ). Together, these results indicate a role for activated CCaMK in cross-signalling between the organogenic and root hair infection thread pathways and a role for SYMRK in the signalling leading to CCaMK activation. In the reciprocal combination of the loss-of-function cytokinin receptor, hit1 , and the autoactive CCaMK in hit1 snf1 double mutants, an excessive infection thread formation comparable to the level observed in hit1 mutants was detected. As previously observed for hit1 mutants [33] , hit1 snf1 mutants show reduced nodulation, whereas organogenesis was absent in uninoculated plants (see Supplementary Table S1 ). The simplest conclusion from these two sets of experiments is that cross-signalling to the root hair infection pathway is CCaMK dependent and that cytokinin signalling mediated by the downstream-functioning snf2 gain-of-function cytokinin receptor was unable to activate the infection thread pathway effectively. See Supplementary Table S1 for the analysis documenting that CCaMK functions upstream of the LHK1 cytokinin receptor. We infer that cross-signalling through CCaMK seems to enhance the efficiency of nodule primordia infection and that cell division alone as in snf2 mutants is insufficient. CYCLOPS was recently suggested to function in the infection pathway and was shown to interact directly with CCaMK [20] , [40] . Our inspection of nodules on cyclops roots transformed with the T265D CCaMK construct confirms the absence of infection and infection threads in cyclops mutants ( Table 1d ), suggesting that CYCLOPS is important for CCaMK cross-signalling from the organogenic to the infection pathway. Previous experiments using a CaMV 35S promoter to drive T265D CCaMK expression resulted in organogenesis beyond the primordial stage, showing that CYCLOPS is dispensable for organogenesis [20] . In our experiments using the cognate CCaMK promoter, this is less obvious and a level of CYCLOPS-dependent back signalling from the infection pathway cannot be excluded. Infection in the absence of NFR1 and NFR5 receptors To determine the requirement for host Nod-factor perception in the intracellular root hair infection thread pathway, double, triple and quadruple mutants of Nfr1 , Nfr5 and SymRK receptors unable to perceive the Nod-factor signal, and/or impaired in downstream signal transduction, were inoculated with M. loti . To our surprise, pink nodules developed in nfr1-1 snf1 and nfr5-2 snf1 double mutants, as well as in nfr1-1 nfr5-2 snf1 , nfr1-1 nfr5-2 symrk-3 snf1 triple and quadruple mutant plants, although at 10- to 20-fold lower frequencies than in snf1 and wild-type plants ( Figs. 4a, h–q and 5 ; Table 1e ). Both normal pink nodules and pink sectored nodules were observed ( Fig. 4b, c, and l–t ). Most plants carrying these nodules displayed dark green leaves and grew, indicating nitrogen fixation in the nodules ( Fig. 5a,b ). Microscopy revealed that infected cells in sectored nodules were not distributed evenly ( Fig. 4m, o and q ) as seen in wild type and most but not all snf1 nodules ( Fig. 4a,h,i ). The invasion process was therefore followed using M. loti strains expressing enhanced green fluorescent protein (eGFP) or lacZ . Using fluorescence and light microscopy, we were unable to detect infection threads in root hairs of nfr1-1 snf1 , nfr5-2 snf1 , nfr1-1 nfr5-2 snf1 and nfr1-1 nfr5-2 symrk-3 snf1 , but thin sections of nodules revealed trans -cellular infection threads in the central nodule tissue ( Fig. 3a–c ). Infection threads were also observed in electon microscopy micrographs ( Fig. 3d–f ). Thin sections of fully or partly infected nodules indicate that these were invaded through infection threads initiated by M. loti entering through cracks at the junctions of nodules and roots, followed by bacterial accumulation in intercellular pockets ( Figs. 3g and 4r–t ). In contrast to the corresponding snf1 double mutants, no infected pink nodules were observed in nfr1-1 snf2 and nfr5-2 snf2 mutants inoculated with M. loti ( Table 1e ). 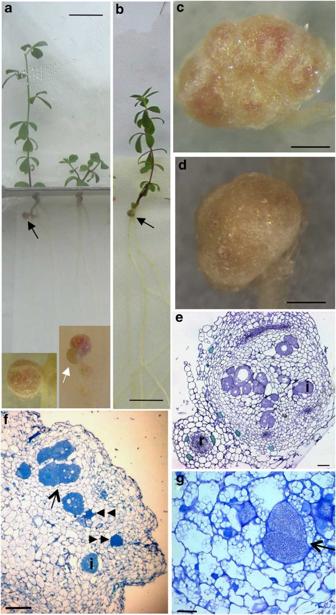Figure 5: Infection of spontaneously induced nodule primordia in the absence of Nod-factor receptors and/or Nod-factor. Development of nitrogen-fixing nodules (black arrows) on (a)nfr1-1snf1and (b)nfr5-2snf1double mutants inoculated withM. loti.Inset: Close-up of infectednfr1-1snf1nodules. White arrow marks uninfected nodule. (c,d) Partially infected spotted nodules on (c)nfr1-1snf1infected bynodAand (d)nfr1-1nfr5-2snf1infected bynodC.(e) Thin section ofnfr1-1snf1 nodAnodule shown in (c), r: root, i: infected cell. (f) Thin section ofnfr1-1nfr5-2 snf1nodule infected bynodC. Double arrowhead: intercellular bacteria, i: infected cell, arrow: newly divided infected cell. (g) Higher magnification of anodC-infected cell in annfr1-1nfr5-2 snf1nodule. Arrow: newly divided infected cell. Size bars (a,b): 1 cm, (c): 20 mm, (d): 500 μm (e) and (f): 100 μm, (g): 10 μm. Figure 5: Infection of spontaneously induced nodule primordia in the absence of Nod-factor receptors and/or Nod-factor. Development of nitrogen-fixing nodules (black arrows) on ( a ) nfr1-1snf1 and ( b ) nfr5-2snf1 double mutants inoculated with M. loti. Inset: Close-up of infected nfr1-1snf1 nodules. White arrow marks uninfected nodule. ( c , d ) Partially infected spotted nodules on ( c ) nfr1-1snf1 infected by nodA and ( d ) nfr1-1nfr5-2snf1 infected by nodC. ( e ) Thin section of nfr1-1snf1 nodA nodule shown in ( c ), r: root, i: infected cell. ( f ) Thin section of nfr1-1nfr5-2 snf1 nodule infected by nodC . Double arrowhead: intercellular bacteria, i: infected cell, arrow: newly divided infected cell. ( g ) Higher magnification of a nodC- infected cell in an nfr1-1nfr5-2 snf1 nodule. Arrow: newly divided infected cell. Size bars ( a , b ): 1 cm, ( c ): 20 mm, ( d ): 500 μm ( e ) and ( f ): 100 μm, ( g ): 10 μm. Full size image Infection in the absence of Nod-factor signalling To further investigate the role of the Nod-factor signal in this alternative intercellular entry process, a set of symrk-3 snf1 , nfr1-1 snf1 and nfr1-1 nfr5-2 snf1 , as well as a har1-3 snf1 hypernodulating mutant, which is impaired in the shoot regulation of nodule numbers by the HAR1 receptor kinase, were inoculated with M. loti nodC or nodA mutants unable to synthesize functional Nod-factors [41] . In symrk-3 snf1 mutants, no infected nodules were observed ( Table 1e ), but interestingly, infections were observed in nfr1-1 snf1 , nfr1-1 nfr5-2 snf1 and snf1 har1 mutants even in the absence of Nod-factor and NFRs. Compared with wild-type and snf1 plants, infection frequencies were reduced 20- to 100-fold ( Table 1e ). Almost all of these pink nodules were sectored and showed irregular morphologies ( Figs. 4d-g , 5c,d ). Using fluorescence and light microscopy and M. loti strains expressing eGFP or lacZ , we were unable to detect infection threads in root hairs or trans -cellular infection threads. Inspection of thin sections of nodules of nfr1-1 snf1 and nfr1-1 nfr5-2 snf1 mutants inoculated with nodC or nodA mutants ( Figs. 3h and 5e,f ) indicates that infection of these nodule primordia occurs through intercellular epidermal entry and shows an anatomy in which only few cells, often only single cells, are infected ( Fig. 5e–g ). These infected cells seem enlarged compared with infected cells in wild-type nodules, suggesting size regulation in wild-type nodules. Infected cells that had recently divided were also observed ( Fig. 5f–g ). Extending the analysis using transmission electron microscopy (TEM), the absence of trans -cellular infection threads was confirmed. TEM micrographs, similar to fluorescence and light microscopy, only reveal intercellularly located bacteria and bacteria inside infected cells ( Fig. 3i ). Among all the sections obtained, two images show sub-cellular structures most likely representing the invasion mechanism operating at the single cell level ( Fig. 3j–l ). The thin section ( Fig. 3j ) shows an intracellular infection that seems to be connected to an adjacent intercellular pocket of bacteria. The TEM micrograph ( Fig. 3k,l ) shows a comparable infection structure. Here, an intercellular pocket of bacteria is located adjacent to an intracellular infection peg that seems to enlarge into a butterfly-shaped release structure containing numerous bacteria. We infer that these expanded intracellular infection pegs are induced by bacterial entry from the intercellular pocket and we propose to call this path for single-cell peg entry. In support of this interpretation, comparable short infection structures originating from intercellular bacteria were observed in lupinoid root nodules [42] , [43] . The results presented here define the components of two parallel pathways facilitating infection thread formation and root nodule organogenesis, respectively ( Fig. 6a ). We have shown that the SYMRK receptor, the two nucleoporins (NUP133, NUP85) and the potassium channels (CASTOR and POLLUX) involved in signal transduction downstream of Nod-factor perception are dispensable for root hair infection thread development and invasion of nodule primordia in an snf1 genetic background. On the other hand, NFRs (NFR1 and NFR5) were required for root hair infection thread initiation, and NAP1 and PIR1 mediating actin rearrangement, together with the putative ubiquitin E3 ligase (CERBERUS), were required for infection thread progression. A simple explanation is an early branching of the NFR and Nod-factor-mediated signal transduction ( Fig. 6a ). NIN, NSP1 and NSP2 transcriptional regulators were required for both infection and organogenesis, supporting a role in both infection thread formation and cortical cell activation. Our results further indicate that calcium spiking by itself is dispensable for infection thread formation, as inactivation of SYMRK, nucleoporins (NUP133, NUP85) and potassium channels (CASTOR and POLLUX) results in an absence of calcium spiking [8] . At the same time, a presumed Ca 2+ activation of CCaMK, as mimicked by the snf1 mutation, seems insufficient for root hair infection thread formation, as functional NFR1 and NFR5 receptors were required for root hair infection thread formation in snf1 . Together this suggests that the NFR receptor-dependent Ca 2+ influx observed in root hairs at high Nod-factor concentration or other, as yet undiscovered, NFR-dependent early responses may be a prerequisite for root hair infection thread formation. Supporting these interpretations, observation of morphological root hair responses in M. truncatula mutants, corresponding to our Lotus symrk , castor / pollux and ccamk mutants, also suggests a separate pathway leading to root hair curling [44] . 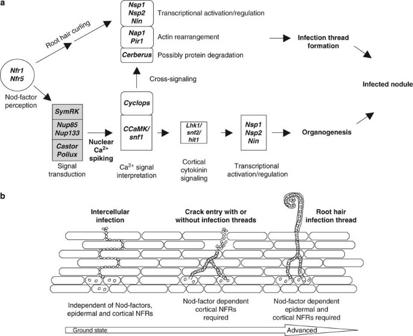Figure 6: Model for evolution of legume nodulation and genes assigned to infection thread and organogenic pathways. (a) Parallel infection thread and organogenic pathways in wild-typeLotus. Cross-signalling through CYCLOPS is indicated. The grey box marks genes that are dispensable for infection thread formation in thesnf1genetic background. (b) Model for molecular evolution of infection pathways in legumes. Intercellular single infection is suggested to be the ground state of rhizobial infection of roots, followed by the crack entry and root hair infection modes. The components of crack entry and single cell infection pathways are less well described and the functional model presented in (a) may only partly represent these infection pathways. Figure 6: Model for evolution of legume nodulation and genes assigned to infection thread and organogenic pathways. ( a ) Parallel infection thread and organogenic pathways in wild-type Lotus . Cross-signalling through CYCLOPS is indicated. The grey box marks genes that are dispensable for infection thread formation in the snf1 genetic background. ( b ) Model for molecular evolution of infection pathways in legumes. Intercellular single infection is suggested to be the ground state of rhizobial infection of roots, followed by the crack entry and root hair infection modes. The components of crack entry and single cell infection pathways are less well described and the functional model presented in ( a ) may only partly represent these infection pathways. Full size image Absence of infection of cyclops primordia after expression of a T265D CCaMK from the CaMV 35S promoter [20] and in our experiments from the CCaMK promoter, together with the reported protein–protein interaction between CCaMK and CYCLOPS, indicates a role for CYCLOPS in cross-signalling between organogenic and infection pathways [20] , [40] . The ineffective invasion in the snf2 mutant background supports this notion and indicates that component(s) responsible for cross-signalling from the organogenic pathway to the infection pathway depend on CCaMK activity while acting upstream of cytokinin responses. In accordance with this interpretation, the hit1snf1 double mutants inoculated with M. loti formed infection threads, whereas ccamk-13 snf2 mutants did not. We suggest that the delayed and the two- to threefold lower infection frequency observed in symrk , nup133 , nup85, castor and pollux mutants within the snf1 background may result from a lack of synchronization between organogenesis and infection, leading to misguidance of infection threads as seen in hit1 mutants [33] . Alternatively, ineffective cross-signalling though autoactive CCaMK proteins may lead to a lower infection frequency. Similarly, lack of synchronization was suggested to explain the delayed nodulation in inoculation of Sesbania plant with a mixture of rhizobial mutant strains [45] . Our results uncover unusual intercellular infection processes in the normally intracellularly root hair-infected Lotus plants ( Fig. 6b ). Intercellular infection and formation of trans -cellular infection threads within the root nodules occurred in the absence of functional NFR1 and NFR5 receptors, although at 10- to 20-fold lower frequencies than in snf1 and wild-type plants. Nevertheless, a comparison of infection thread formation induced by wild-type M. loti and nodC mutants shows that synthesis of the bacterial Nod-factor was required for the effective development of these trans -cellular nodule infection threads. The mechanism involved in such a cortical perception is unknown, but involvement of one or more of the 15 additional receptor kinases belonging to the Lotus NFR1 and NFR5 families is conceivable [46] . Six of these family members, Lys2, Lys3, Lys7, Lys12, Lys15 and Lys20 , were expressed mainly in root and root nodules [46] and are thus candidates for the cortical receptor or receptor components. Involvement of alternative epidermal or cortical NFRs is supported by observations in Sesbania , in which root hair infection was stringently dependent on an intact Nod-factor structure, whereas crack entry was less stringently controlled [47] , [48] but still dependent on continuous Nod-factor synthesis for effective invasion [49] . Furthermore, the suggested cross-signalling through CCaMK and CYCLOPS interaction also seems to be required for nodule infection thread formation following the intercellular infection mode. Absence of intercellular infection in nfr1-1 snf2 , nfr5-2 snf2 , ccamk-13 snf2 and cyclops snf1 mutants concurs with this interpretation, as does the recent observation of impaired infection thread progression following RNA-mediated interference knockdown of CCaMK in Sesbania [50] . Intercellular infection of single cells as observed in, for example, nfr1 nfr5 snf1 mutants inoculated with the bacterial nodC mutant may constitute the ground state of bacterial invasion mobilized during evolution of nodulation. This intercellular process was approximately 20- to 100-fold less effective than normal root hair invasion. Symbiosomes were observed in infected cells, indicating that endocytosis occurred in the absence of Nod-factor and NFR1 and NFR5 receptors. Endocytosis in the apparent absence of local Nod-factor synthesis in cortical infection threads was also observed in mixed inoculation of Sesbania [49] . In this context, the lack of infected nodules observed in symrk snf1 double mutant plants inoculated with nodC and nodA mutant strains is puzzling. This may suggest that the SYMRK receptor would be necessary for single cell infection in contrast to infection through infection threads. However, the low level of infection by nodC and nodA mutant strains observed on nfr1 nfr5 snf1 mutants cautions such a conclusion on the basis of negative results. Considering our positive results with nodC and nodA infection of nfr1 nfr5 snf1 mutants, we hypothesize that a capacity for direct intercellular infection may constitute an ancient invasion path that evolved at the emergence of the legume family or maybe at the emergence of the eurosid I clade containing all nodulating plants. Division of primary infected single cells would conceivably lead to the fully infected Nod-factor-independent nodulation observed in Aeschynomene- type nodules [1] , [51] . In a subsequent evolutionary step, the Nod-factor and cortical NFR-dependent crack entry and subsequent cortical infection thread propagation of invasion could have been established. The most highly evolved state envisaged is the root hair infection mode. This infection mode required Nod-factor, epidermal NFR1 and NFR5 receptors, and is predicted to also involve cortical NFRs with less stringency than NFR1 and NFR5 receptors. The ability of Sesbania to switch between a root hair infection mode requiring Nod-factor decorations and a crack entry mode less dependent on Nod-factor structure [48] supports our interpretation, as does the infrequent and delayed infection of nodules in a root hairless mutant [52] and rare events in flooded Lotus spp [53] . Overall, this model postulates an evolutionary process in which the advanced root hair infection bestowed a set of legume hosts with a tighter and more selective control of bacterial passage through the epidermis ( Fig. 6b ). Our observations also suggest that alternative invasion modes have been maintained during evolution and that they are not mutually exclusive. Presence of different infection modes in Sesbania , Chamaecrista [1] , and both a Nod-factor-dependent and a Nod-factor-independent mechanism for nodulation in Aeschynomene sensitiva [51] , is in accordance with these notions. On this basis, we propose that taking non-exclusive infection modes into account may contribute to resolving some of the difficulties in aligning nodule evolution and the legume phylogeny [1] . Further studies of the direct infection pathway(s) will not only impact biotechnological applications and improve our understanding of plant–microbe interactions but may be key to elucidate the evolution of symbiosis. Plant material The L. japonicus mutants used in this study are all in an ecotype Gifu B-129 background [54] . Bacterial strains For details on M. loti strains, see Supplementary Table S2 . The identity of bacteria in selected, infected nodules was confirmed by re-isolation of bacteria from surface-sterilized nodules, followed by genotyping by specific PCR. For primers, see Supplementary Table S3 . Double mutants and plant genotyping Double, triple and quadruple mutants were obtained by crossing, followed by genotyping of offspring plants. Similarly, the genotypes of mutant plant lines in individual experiments were verified using allele-specific PCR and/or sequencing of PCR-amplified genomic fragments (for primers and conditions, see Supplementary Table S4 ). The non-nodulating mutants used to establish crack entry, single cell infection and cross-signalling mechanisms (summarized in Fig. 6a,b ) carry stable mutations caused by insertion of LORE1 or LORE2 retrotransposons ( symrk-1 , symrk-3 , nfr5-2) , a deletion ( ccamk-13) or a premature stop codon ( nfr1-1) . See Supplementary Table S4 for a full list of genotypes of the mutants used in this study. DNA techniques The constitutively active T265D variant of the Lotus CCaMK gene driven by the native CCaMK promoter was constructed using overlap extension PCR for site-directed mutagenesis of the wild-type CCaMK construct [17] and conventional cloning techniques. The construct complements the nodulation defect in Lotus ccamk mutants [17] and causes spontaneous nodulation in the absence of rhizobia. Transgenic hairy roots carrying CCaMKT265D or control wild-type CCaMK genes were produced through A. rhizogenes transformation [9] . Plant growth conditions Seeds of wild type and mutants were surface sterilized for 20 min in a solution of 0.5−1.0% sodium hypochlorite and grown in a 16/8 h day/night regime of 21/16 °C for up to 7 weeks in square Petri dishes on solid 1/4 B&D slants without nitrate, or in Magenta containers (Sigma) on a substrate of Leca (Optiroc) and Vermiculite (3:1 mixture) supplemented with 75 ml of 1/4 B&D medium without nitrate. On plates, the plant roots were shielded from light by using a metal comb fitting the Petri dish and inserting the lower half of the Petri dish into a rack. Plants were grown with or without inoculation with M. loti strains (see below). Nodule counts Red and white nodules/nodule primordia were counted and photographed using a Zeiss Discovery V8 stereomicroscope. Infection thread analysis To visualize infection threads, roots were inoculated with M. loti expressing lacZ or eGFP reporter genes. Each seedling was inoculated with 150−400 μl (OD600 ∼ 0.01 to 0.02) of M. loti expressing the relevant reporter gene and infection threads were visualized at selected time points after inoculation by staining for β-galactosidase activity [8] After clearing in 30% lactic acid, the roots were mounted on glass slides in glycerol and observed with a bright field Zeiss Axioplan microscope with ×10, ×20 or ×40 objectives, equipped with DIC optics. For eGFP-expressing bacteria, intact roots were mounted on slides in deionized water and observed directly with a Zeiss fluorescence microscope with standard FITC filters. Images were taken with a Zeiss LSM 510 Meta confocal microscope, with excitation at 488 nm, and a BP 505−530 emission filter. Images were recorded with Axiovision software. The number of infection threads was recorded either per root for short roots or per cm root for older, longer roots. Roots from at least two different plants were scored for each genotype and between 10 and 80 cm roots were inspected for each genotype. The number of infection threads in thin sections was counted in two representative sections of 10 different nodules for each plant genotype. Microscopy Nodules were prepared for light and TEM coupled with immunogold labelling with the rat monoclonal antibody MAC236 [42] and infection threads from all genotypes were labelled. Nodules that had been fixed in 2.5% glutaraldehyde in 0.1 M sodium cacodylate (pH 7.0) overnight at 4 °C were dehydrated in an ethanol series, and embedded in LR White acrylic resin (Agar Scientific). Semithin sections (1 μm) were taken for light microscopy and ultrathin (70 nm) sections were taken for TEM using a Leica UCT ultramicrotome. The semithin sections were collected on glass slides and stained with 0.1% toluidine blue, whereas the ultrathin sections were collected on pioloform-coated nickel grids and immunogold labelled with the MAC236 antibody. The sections were incubated for 2 h in MAC236 (diluted 1:10), followed by 30 min incubation in an anti-rat secondary antibody raised in rabbit (diluted 1:400) (Southern Biotechnology), and then for 1 h in 15 nm goat anti-rabbit gold (GE Healthcare) (diluted 1:100). The ultrathin sections were then stained with uranyl acetate for 10 min before being viewed and digitally photographed using a JEM 1400 transmission electron microscope (JEOL). Note that bacteria inside Lotus infection threads may seem crenellated [53] . How to cite this article: Madsen L.H. et al . The molecular network governing nodule organogenesis and infection in the model legume Lotus japonicus . Nat. Commun. 1:10 doi: 10.1038/ncomms1009 (2010). Copyright: © 2010 Madsen, L.H. et al . This is an open-access article distributed under the terms of the Creative Commons Attribution License, which permitsunrestricted use, distribution and reproduction in any medium, provided the original author and source are credited.